Frequent new particle formation over the high Arctic pack ice by enhanced iodine emissions 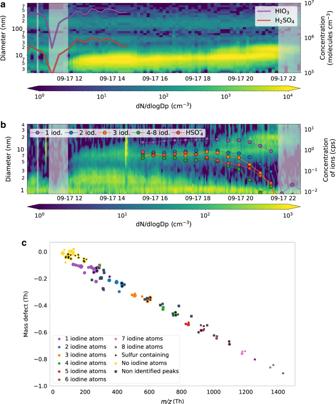Fig. 1: New particle formation mechanisms over the pack ice shown for 17 September 2018. aEvolution of particle size distribution; also shown are the iodic and sulfuric acid monomer concentration measured with a nitrate chemical ionization mass spectrometer.bNegative-ion size distribution from neutral cluster and air ion spectrometer measurements and naturally charged sulfuric acid and iodine clusters measured with the negative atmospheric pressure interface time of flight (APi-TOF) mass spectrometer. The legend indicates the number of iodine atoms per cluster where clusters with the same number of iodine atoms were summed up. The concentration is given in counts per second (cps). Grey shaded areas indicate periods with fog (here associated to a visibility below 2 km).cMass defect plot of the negatively charged ions measured with the APi-TOF. The size of the markers is proportional to the logarithm of the concentration. The iodine clusters reported in the mass defect plot are the same as shown in the bottom panel of Fig.1b. Squares indicate peaks for which it has not been possible to unambiguously identify their chemical composition, however their mass defect is compatible with iodine containing species. In the central Arctic Ocean the formation of clouds and their properties are sensitive to the availability of cloud condensation nuclei (CCN). The vapors responsible for new particle formation (NPF), potentially leading to CCN, have remained unidentified since the first aerosol measurements in 1991. Here, we report that all the observed NPF events from the Arctic Ocean 2018 expedition are driven by iodic acid with little contribution from sulfuric acid. Iodic acid largely explains the growth of ultrafine particles (UFP) in most events. The iodic acid concentration increases significantly from summer towards autumn, possibly linked to the ocean freeze-up and a seasonal rise in ozone. This leads to a one order of magnitude higher UFP concentration in autumn. Measurements of cloud residuals suggest that particles smaller than 30 nm in diameter can activate as CCN. Therefore, iodine NPF has the potential to influence cloud properties over the Arctic Ocean. The Arctic is warming at least twice as fast as the global average (Arctic amplification) [1] , [2] , particularly during autumn and winter [3] . Model studies have identified several local and remote drivers that contribute to the accelerated warming. State-of-the-art climate models are still unable to accurately represent local Arctic processes. This is particularly true for clouds and their radiative properties [3] , [4] . The presence or absence of a cloud over the pack ice makes a significant difference for the surface energy budget and is expected to impact the thickness and extent of sea ice [5] . Cloud formation in the central Arctic Ocean can be limited by the availability of cloud condensation nuclei (CCN) [6] . Under this CCN-limited cloud regime, a small increase in the CCN concentration can lead to a pronounced increase in surface warming due to the longwave cloud forcing. Hence, understanding the sources and evolution of particles in the central Arctic Ocean is crucial to modeling the CCN population and cloud formation correctly. Previous measurements in the region have revealed a number of CCN sources, including secondary marine organic particles, primary marine emissions like sea salt and organic aerosol, long-range transported continental emissions and their down-mixing into the marine boundary layer from aloft [7] , [8] , [9] , [10] . Continental influence may make up about one-third of the non-refractory accumulation mode particles [7] , highlighting the importance of regional and local Arctic sources which are not yet well constrained. This is particularly true for new particle formation (NPF) and Aitken mode particles since the online instrumentation capable of characterizing their chemical composition in situ has become available only recently [11] , [12] . A recent modeling work suggested that NPF may contribute to a large fraction of the high Arctic CCN number concentration [13] . However, no information was provided about the source region of these newly formed particles and none of the models currently includes iodine nucleation. Thus, the actual contribution of local NPF to the Arctic CCN budget remains highly uncertain. Nucleation mode particles have been observed over the pack ice since the first International Arctic Ocean Expedition in 1991 [14] , [15] , [16] , [17] , and are typically associated with prolonged air mass residence time over the pack ice, suggesting the influence of a source within the pack ice [18] . However, the source of these newly formed particles has not been identified [16] , [17] . Measurements around the Arctic marginal ice zone (MIZ) have attributed NPF to sulfuric acid, ammonia, marine organics [19] , [20] and in a few cases to iodine [21] , [22] , [23] . While these studies provide valuable information about Arctic NPF they cannot be directly extrapolated to the central Arctic Ocean, which is characterized by a much lower concentration of gas precursors compared to the MIZ [24] . By deploying a real-time mass spectrometer [11] , [12] and various particle counters and sizers we have identified iodic acid (HIO 3 ) as the main driver for the frequent NPF events occurring over the central Arctic Ocean during August and September, the expedition period. Data were collected during the Microbiology–Ocean–Cloud-Coupling in the High Arctic (MOCCHA) campaign as part of the Arctic Ocean 2018 expedition on board the Swedish icebreaker (I/B) Oden (Supplementary Fig. 1 ). Iodine drives NPF A typical NPF event is illustrated in Fig. 1a . Iodic and sulfuric acid (H 2 SO 4 ) increase before 10:00 (all times given in UTC) leading to the production of small particles as evident from the negative-ion number size distribution. During the passage of a small patch of fog, both the concentration of the acids and the newly formed particles are strongly reduced but increase again afterwards. On the regional scale particles have already grown to 3–7 nm size. While HIO 3 reaches a concentration of >8 × 10 6 molecules cm −3 , the sulfuric acid concentration remains six to ten times lower. The negatively charged clusters are composed of iodine oxides with a maximum of eight iodine atoms per cluster, whereas the largest pure sulfuric acid cluster detected is only the trimer (mass defect plot in Fig. 1b ). Mixed clusters are also detected containing a maximum of two sulfur and up to eight iodine atoms. The chemical composition of the pure iodine clusters is typically H 0−4 O x I y with an oxygen to iodine ratio between 2.5 and 3. This closely resembles the first measurements of coastal HIO 3 nucleation performed in Mace Head (Ireland) [21] , pointing towards a similar nucleation mechanism. The oxygen to iodine ratio is also in agreement with previous laboratory and modeling iodine NPF studies [25] , [26] ; the full list of both neutral and charged iodine clusters is reported in Supplementary Tables 1 and 2 . Fig. 1: New particle formation mechanisms over the pack ice shown for 17 September 2018. a Evolution of particle size distribution; also shown are the iodic and sulfuric acid monomer concentration measured with a nitrate chemical ionization mass spectrometer. b Negative-ion size distribution from neutral cluster and air ion spectrometer measurements and naturally charged sulfuric acid and iodine clusters measured with the negative atmospheric pressure interface time of flight (APi-TOF) mass spectrometer. The legend indicates the number of iodine atoms per cluster where clusters with the same number of iodine atoms were summed up. The concentration is given in counts per second (cps). Grey shaded areas indicate periods with fog (here associated to a visibility below 2 km). c Mass defect plot of the negatively charged ions measured with the APi-TOF. The size of the markers is proportional to the logarithm of the concentration. The iodine clusters reported in the mass defect plot are the same as shown in the bottom panel of Fig. 1 b. Squares indicate peaks for which it has not been possible to unambiguously identify their chemical composition, however their mass defect is compatible with iodine containing species. Full size image The sulfuric acid neutral monomer concentration is more than two orders of magnitude too low for binary NPF [27] , while ternary sulfuric acid NPF with bases can be ruled out by the absence of clusters containing ammonia or amines in the negative-ion mass spectrum [27] , [28] . Furthermore, the continuous growth of the negative-ion size distribution from the ion cluster band (0.8–1.2 nm) is clear evidence that ultrafine particles (UFP) (defined here as particles with diameter D < 15 nm) are produced by secondary particle formation. We did not find any evidence that UFP were produced by a primary mechanism as hypothesized previously [29] . During this campaign, we detected 11 major NPF events over the pack ice in total, all driven by HIO 3 with no important contribution from sulfuric acid or other compounds. All the events were characterized by a continuous growth of the negative ions from the cluster band into larger sizes, whereas no growth of the positive ions was observed. This indicates that ion-induced NPF is purely negative as expected for HIO 3 which has a very low proton affinity [21] . However, we were not able to quantify the importance of ion-induced compared to neutral NPF for our set of measurements. A list of the events with the relative particle size distributions (PSD) and negative-ion spectra is reported in Methods section (Supplementary Fig. 2 ). Iodic acid sources, sinks, and variability The 2-month time series of the HIO 3 concentration shows a clear and steady increase around the end of August (Fig. 2a ), leading to an increase of the UFP concentration by more than one order of magnitude from summer (August) to autumn (September) (Fig. 2b ). The covariation between HIO 3 and UFP (Fig. 2a ) highlights the important role of HIO 3 and suggests that there were no other important sources of UFP over the pack ice during this period. The aggregated summer/autumn average comparison shows that sulfuric acid and methanesulfonic acid (MSA) are much less enhanced in autumn compared to HIO 3 (Supplementary Fig. 3 ). Fig. 2: Factors controlling iodic acid concentration and NPF over the pack ice in the central Arctic Ocean. a Daily box and whiskers plot of iodic acid, where the box extends from the first quartile (Q1) to the third quartile (Q3) with a line indicating the median. The whiskers are set to 1.5*[Q3–Q1]. The boxes are color-coded with the daily mean air temperature measured from the upper deck of the ship (roughly 25 m above sea level). The continuous green line shows the ozone concentration (axis on the right). b Daily box and whiskers plot of the ultrafine particle concentration (UFP), particles with a diameter between 2.5 and 15 nm. The continuous line shows the near-surface air temperature, with values lower than −2 °C colored in blue and above in yellow (axis on the right). c Iodic acid concentration during autumn as a function of visibility, dots indicate the median and the shaded area the interquartile range [Q3–Q1]. d Iodic acid concentration box and whiskers plot for different conditions during the autumn period. In particular, we report values for the entire autumn period, during fog (visibility below 2 km) and during NPF events. e Iodic acid data as a function of dry deposition velocity ( v d ), boundary layer height ( h ) and condensation sink (CS). Iodic acid data correspond only to clear conditions (visibility > 4 km) and periods when steady-state conditions could be assumed. Eleven steady-state periods are given by differently colored symbols. The colored lines represent different emission rates ( E ) based on our model. Full size image This clear regime change seems to be associated with a much weaker source of iodine during summer. Air mass back trajectories do not show a systematic difference in source region between summer and autumn (Supplementary Fig. 4 ). The fact that high concentrations of HIO 3 were detected for several days continuously and over a large latitudinal range (from 89°N to 82°N approximately) points towards a pack ice-wide source rather than a local phenomenon. The transition from summer to autumn coincides with dropping temperatures and the start of the freeze-up period (sea ice formation). We identified the freeze onset as 28 August based on the running mean of the near-surface air temperature [30] . However, the freeze-up occurs over several days with multiple freezing and melting cycles. The near surface temperature dropped below zero around 13 August and then remained between −2 and 0 °C for several days. This intermediate phase corresponds to a steady increase in the HIO 3 concentration. Between 27 and 28 August the near surface temperature shows a step decrease to below −2 °C (Fig. 2b ), which corresponds to the freeze-up onset and to the occurrence of the first NPF event. Previous studies have shown that iodine can be produced by microalgae below sea ice and transported via brine channels or cracks to the atmosphere [31] , [32] . Abiotic mechanisms can also release iodine from the snowpack and frozen saline surfaces via condensed phase reactions [33] , [34] , [35] , [36] , [37] . Concurrently with HIO 3 we also observed a marked increase of the ozone concentration (Fig. 2a ), similar to measurements at Alert, in the Canadian Arctic [38] . A higher ozone concentration can enhance the emission of iodine from seawater and frozen saline surfaces [35] , [37] , [39] , consistent with our observations. Therefore, we hypothesize that the increase in HIO 3 concentration and NPF frequency are linked to both, the formation of new sea ice and the increase in the ozone concentration. However, the individual contributions of these two processes cannot be disentangled with our set of measurements. Dedicated in situ measurements in the central Arctic Ocean are required to investigate these phenomena and precisely identify their contributions to the increased iodine emissions. Importantly, while at Arctic land-based observatories further south the occurrence of nucleation mode particles has generally been associated with biological activity in melting sea ice regions, primarily between May and August [22] , [40] , [41] , NPF has so far never been associated with the freeze onset. The HIO 3 concentration and the occurrence of NPF are regulated by local meteorology. In the central Arctic Ocean fogs and clouds are the dominant sink for these species since the low aerosol background concentration provides a very low condensation sink (CS) on the order of 10 −5 –10 −4 s −1 (Supplementary Fig. 5 ), more than one order of magnitude lower than most clean continental sites [42] . Because of the absence of any other important sink, a tenuous fog with visibility just below 4–5 km reduces HIO 3 enough to prevent NPF (Fig. 2c and d ). During clear conditions the HIO 3 variability can be largely explained through the interplay of the surface mixed layer height ( h ), the CS and the dry deposition velocity of the gas ( v d ). We have developed a simple model to combine these three factors and an emission rate ( E in atoms cm −2 s −1 ) of iodine that is assumed to be constant over the course of an event (details are given in the Methods section). The concentration of HIO 3 at the steady-state can be described by 
    [ log _10([ HIO_3]) = log _10E - log _10(v_d + h ·CS) ]
 (1) The emission rate E is a net term that accounts for the emission of iodine from the surface and its conversion into HIO 3 which may occur via several intermediate reactions [21] , [43] . We have identified 11 periods satisfying a steady-state assumption. 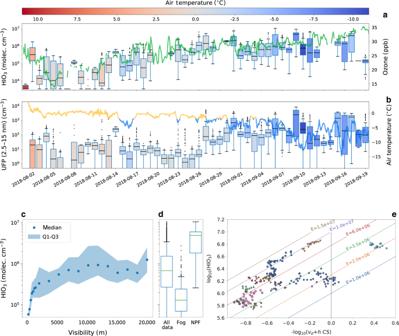Fig. 2: Factors controlling iodic acid concentration and NPF over the pack ice in the central Arctic Ocean. aDaily box and whiskers plot of iodic acid, where the box extends from the first quartile (Q1) to the third quartile (Q3) with a line indicating the median. The whiskers are set to 1.5*[Q3–Q1]. The boxes are color-coded with the daily mean air temperature measured from the upper deck of the ship (roughly 25 m above sea level). The continuous green line shows the ozone concentration (axis on the right).bDaily box and whiskers plot of the ultrafine particle concentration (UFP), particles with a diameter between 2.5 and 15 nm. The continuous line shows the near-surface air temperature, with values lower than −2 °C colored in blue and above in yellow (axis on the right).cIodic acid concentration during autumn as a function of visibility, dots indicate the median and the shaded area the interquartile range [Q3–Q1].dIodic acid concentration box and whiskers plot for different conditions during the autumn period. In particular, we report values for the entire autumn period, during fog (visibility below 2 km) and during NPF events.eIodic acid data as a function of dry deposition velocity (vd), boundary layer height (h) and condensation sink (CS). Iodic acid data correspond only to clear conditions (visibility > 4 km) and periods when steady-state conditions could be assumed. Eleven steady-state periods are given by differently colored symbols. The colored lines represent different emission rates (E) based on our model. Figure 2e shows the dependence of HIO 3 on ( v d + h CS) for each period with differently colored symbols and expected linear trends by our model for different values of E . Data from each period was grouped around a given emission factor with some variability that probably reflects the simplicity of our model. Overall, the emission factor median and interquartile range (IQR) are equal to 5.0 [3.2–7.6] × 10 6 iodine atoms cm −2 s −1 with the full data distribution being shown in Supplementary Fig. 6 . In Supplementary Fig. 7 , we show the fairly good agreement of a simulation of the HIO 3 concentration for a high and a low emission case scenario, corroborating our model and the underlying assumptions. Despite its simplicity, our model can explain a large fraction of the HIO 3 variability with emission rates ranging between 1.5 and 15.4 × 10 6 iodine atoms cm −2 s −1 (two standard deviations of the mean). This range is likely a lower limit estimate of the real emission rates as not all iodine atoms would be converted into HIO 3 , however, it represents a valuable approach on which Earth system models could build to implement iodine NPF in the central Arctic Ocean. Ultrafine particle growth and survival This newly identified nucleation mechanism represents a massive source of aerosol particles for the central Arctic Ocean, which is usually characterized by extremely low aerosol concentrations [10] , [20] . For example, during this expedition, the median and IQR concentration of particles above 30 nm is 26 [10–48] cm −3 and the CCN concentration at 0.3% supersaturation (SS) is 17 [6–33] cm −3 (Supplementary Fig. 5 ). However, the relevance of NPF for the local cloud budget depends on the probability that newly formed particles grow to larger sizes where they can act as CCN. The fate of newly formed particles is determined by their growth-to-loss rate ratio, with their growth being controlled by the concentration of condensable vapors and their loss by coagulation with other surfaces (i.e. pre-existing aerosol or fog droplets). Given the low particle concentration UFP are mainly lost through coagulation with fog droplets. Typically, meteorological conditions are very variable as shown in Fig. 3b . The measurement of the newly formed particles and their growth is rapidly interrupted, when the visibility drops below a few  km. Fog in the central Arctic Ocean is characterized by a low number of droplets (usually below 30–50 cm −3 during our campaign) due to CCN limitation. While the nucleating species with their high diffusivity rapidly disappear (Fig. 3b ), UFP with a relatively long lifetime of ~2.5 h for a 5 nm particle are not expected to disappear as fast as observed (Supplementary Fig. 8 ). Our interpretation is that longer-lived patches of fog are advected to the observation point (the ship). Depending on the history of the foggy air mass, UFP may have been partially taken up by the fog droplets at the time of arrival or NPF was even inhibited because of the fast removal of HIO 3 . This explanation is consistent with the fact that, after passage or dissipation of the fog, a UFP mode re-appeared, suggesting substantial continuity with the mode before the fog. This indicates that the fog is a spatially small-scale phenomenon, and that NPF was occurring on a larger scale with an estimated minimum air mass diameter of 160 km for this event (see Methods section). From the time trend of the PSD it is quite evident that the growing mode disappears and reappears at least three times during this event as well as during the following event in association with fog patches. Fig. 3: Ultrafine particle growth and losses. a Particle size distribution (PSD) measured with a neutral cluster and air ion spectrometer (NAIS) with the indication of the fitted mode diameter used for growth rate calculation. The black hatched region indicates a period influenced by pollution from the ship. b Concentrations of iodic and sulfuric acid together with visibility. Grey shaded areas indicate fog periods. c Growth rate (GR) measurements for the entire campaign as a function of the mean diameter mode during the event. The blue marker shows the measured growth rate obtained by fitting the mode diameter (the error bars represent the 95% confidence intervals from the fitted slope). The bar plot shows the estimated growth rate based on the mean mode diameter and the concentration of sulfuric and iodic acid [44] . The black lines are the error bars due to the uncertainty of sulfuric and iodic acid concentration. The red dashed bars show the predicted growth rate when considering also the charge enhancement factor (EF) derived from Stolzenburg et al. [45] Since for the last three events iodic and sulfuric acid measurements are not available, we report only the measured growth rates. Full size image Because of the long lifetime of UFP they can grow continuously for several hours reaching 15–20 nm in size, despite the low growth rates that range between 0.2 and 1.2 nm h −1 with a median and IQR of 0.5 [0.4–0.6] nm h −1 (Fig. 3c ). Assuming kinetic condensation [44] we calculated the fraction of the growth attributable to iodic and sulfuric acid for all the events of the campaign with a clearly detectable growth (details in Methods section). In the majority of the cases more than 50% of the growth can be attributed to HIO 3 alone (Fig. 3c ). Sub-10 nm aerosol growth can be enhanced by dipolar interactions [45] , [46] but the enhancement factor (EF) for HIO 3 is not known. By applying the sulfuric acid EF [45] most of the growth could be explained within uncertainty by HIO 3 alone (Fig. 3c ). Moreover, we did not consider other iodine oxides that can partition into the particle phase [43] and contribute to the growth because we were not able to quantify their concentration. However, these compounds probably account for another fraction of the growth. There are, however, two events (cases 3 and 5 in Fig. 3c ) where only a small fraction of the growth could be explained. For these cases some other compounds must have contributed to the growth, most likely organics that were not oxygenated enough to be detectable with a nitrate CIMS [47] . While no gas phase measurement is available during the last event, the required HIO 3 concentration to explain such a large growth would be higher than any value measured during the campaign. The more a newly formed particle grows the longer it survives (a 30 nm particle has a 10 times longer lifetime compared to a 10-nm particle) and the more likely it is that it can act as CCN. In summary, HIO 3 is not only vital for the formation of new particles above the pack ice but also for their growth and hence for their survival. NPF contribution to the CCN budget Since the growth rate of newly formed particles is generally below 1 nm h −1 it takes them several hours to days to reach a size where they can act as CCN (e.g. 30 nm at 1% SS [48] ). However, the variability of fog occurrence and the frequent air mass and weather changes reduce the probability of observing the same aerosol population growing up to CCN size [49] . Low-level clouds in the Arctic are generally characterized by an SS of 0.3% which would not be sufficient to activate 20–40 nm particles [50] . However, it has been indirectly shown that droplets often form on particles smaller than 50 nm [50] , [51] . 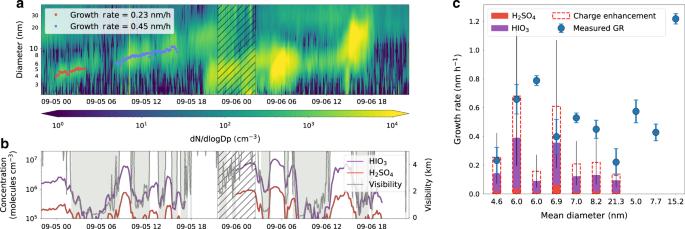Fig. 3: Ultrafine particle growth and losses. aParticle size distribution (PSD) measured with a neutral cluster and air ion spectrometer (NAIS) with the indication of the fitted mode diameter used for growth rate calculation. The black hatched region indicates a period influenced by pollution from the ship.bConcentrations of iodic and sulfuric acid together with visibility. Grey shaded areas indicate fog periods.cGrowth rate (GR) measurements for the entire campaign as a function of the mean diameter mode during the event. The blue marker shows the measured growth rate obtained by fitting the mode diameter (the error bars represent the 95% confidence intervals from the fitted slope). The bar plot shows the estimated growth rate based on the mean mode diameter and the concentration of sulfuric and iodic acid44. The black lines are the error bars due to the uncertainty of sulfuric and iodic acid concentration. The red dashed bars show the predicted growth rate when considering also the charge enhancement factor (EF) derived from Stolzenburg et al.45Since for the last three events iodic and sulfuric acid measurements are not available, we report only the measured growth rates. We provide here direct evidence that particles in the 20–40 nm size range activate as CCN in Arctic fog when the concentration of larger aerosols is low enough; this suggests that iodine NPF may be a relevant CCN source in the region. One example is the activation of Aitken mode particles on 6 September (Fig. 4 ), the second part of the event described in Fig. 3 . We compare the properties of the dry PSD with measurements of cloud particle residuals obtained with a counter-flow virtual impactor (CVI) inlet. 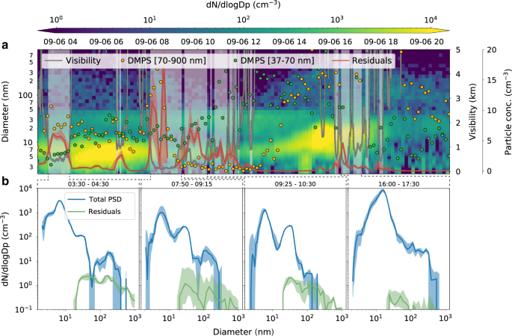Fig. 4: Activation of Aitken mode particles in fog. aParticle size distribution, visibility, particle concentrations in two different size ranges (37–70 and 70–900 nm, representing the larger tail of the Aitken mode and the accumulation mode, respectively) and the total droplet residual concentration (the solid line is the 10-min median and the shaded area the interquartile range, IQR). Grey shaded areas indicate fog periods.bMedian (solid line) and IQR (shaded area) particle and residual size distribution for the four different fog periods during the event. The cloud residuals distribution is based on measurements with a differential mobility particle sizer (DMPS) behind a counter flow virtual impactor inlet. Figure 4a shows the PSD of the entire aerosol population with diameters D from 2 to 900 nm, overlaid with the particle concentrations in two different size ranges (37 < D < 70 nm and 70 < D < 900 nm), the concentration of cloud residuals, and the visibility. During the fog period from 08:00 to about 12:00, the accumulation mode particle concentration dropped below 1 cm −3 after 09:00. This is a clear indication that smaller particles act as CCN to sustain the fog. The residual number concentration matches the integrated aerosol concentration with diameters above 37–44 nm (the size of a diameter size bin), providing an upper limit estimate on the activation diameter. The real activation diameter is likely smaller given that this CVI only sampled droplets larger than 7.8 µm and a fraction of the droplets was persistently smaller than this threshold (Supplementary Fig. 8 ). Based on the CCN and size distribution measurements for this event (Supplementary Fig. 9 ) we estimate that an SS close to 1% is required to activate particles in this size range. It is conceivable that such high SS can occur due to the small total number of droplets such that excess water vapor is not depleted as quickly as in more accumulation mode-rich environments. Fig. 4: Activation of Aitken mode particles in fog. a Particle size distribution, visibility, particle concentrations in two different size ranges (37–70 and 70–900 nm, representing the larger tail of the Aitken mode and the accumulation mode, respectively) and the total droplet residual concentration (the solid line is the 10-min median and the shaded area the interquartile range, IQR). Grey shaded areas indicate fog periods. b Median (solid line) and IQR (shaded area) particle and residual size distribution for the four different fog periods during the event. The cloud residuals distribution is based on measurements with a differential mobility particle sizer (DMPS) behind a counter flow virtual impactor inlet. Full size image The activation of small Aitken mode particles is directly evident from the residual size distribution measured with a DMPS behind the CVI. Figure 4b shows the average residual size distributions for four different fog periods during the same day, and, as a reference, the corresponding average size distributions of the total aerosol population. In all four cases, there is a clear and consistent presence of Aitken mode particles in the cloud residuals smaller than 30 nm. It is important to note that iodine NPF is not the only source contributing to the total Aitken mode aerosol population over the pack ice. Long-range transport of secondary particles formed in more biologically productive regions, such as the MIZ, may also be an important source [20] . As such, there is a clear need for dedicated studies on the sources of Aitken mode particles and their role for the Arctic CCN budget to quantitatively assess the importance of this newly identified NPF mechanism. The source of NPF over the pack ice in the central Arctic Ocean has been elusive for almost 30 years. This study provides direct molecular evidence that iodine is the driver of NPF in August and September over the central Arctic Ocean while we find no evidence that UFP were produced by a primary mechanism as previously hypothesized [29] . We also show for the first time that the HIO 3 concentration over the pack ice increases steadily towards the end of August. We hypothesize that this trend is related to the formation of new sea ice and to the increase of boundary layer ozone. This is in line with observations at Alert, Canada, between 1980 and 2006, where, during autumn, higher ozone concentrations and a second peak of iodine in the aerosol was found (the first being in spring) [38] , [52] . Their seasonality of the iodine concentrations is remarkably similar to our HIO 3 trend indicating that our observations are not unique to the 2018 season (Supplementary Fig. 10 ). Terminology note The beginning of the autumn season in the Arctic is generally associated with colder temperature and the formation of new sea ice, in contrast to the summer melt season [53] . For this reason and to be clear, in our work, we consistently refer to these two periods as summer and autumn. However, because our measurements cover August and September specifically, our findings are representative of the summer to autumn transition and cannot be directly extrapolated to the full Arctic summer and autumn seasons. Campaign description Data were collected during the MOCCHA campaign as part of the US-Swedish expedition Arctic Ocean 2018 on board the Swedish I/B Oden in August and September 2018 with more than 4 weeks of ice-drift operation at latitudes higher than 88°N (Supplementary Fig. 1 ). Instrumentation and measurements Aerosol and cloud-related measurements were conducted on the 4th deck of I/B Oden inside two different containers. Three different inlets were used for this study, a NPF inlet designed to minimize diffusional losses with a short residence time, a whole air inlet sampling the entire aerosol population (interstitial and activated) and a CVI inlet sampling only cloud droplets and ice crystals larger than 7.8 µm (more details are provided below). HIO 3 , sulfuric acid, and MSA were measured using a nitrate chemical ionization mass spectrometer [54] . These molecules are detected both as deprotonated species and clustered with the nitrate monomer. The instrument was calibrated after the campaign for sulfuric acid as described in Kürten et al. [55] , the same calibration constant was assumed also for HIO 3 and MSA. This assumption is motivated by the fact that these three molecules have a lower proton affinity compared to nitric acid and the ionization proceeds at the kinetic limit. Diffusion losses in the inlet were corrected using the diffusion constant of sulfuric acid [56] . The uncertainty in the determination of these compounds in well-controlled experiments is usually estimated to be −30%/+50% [45] . However, it is common to extend the uncertainty to −50%/+100% for field measurements in order to account for the intrinsic variability of field conditions that cannot be quantified. We decided to use the larger uncertainty although it is likely to be an overestimation. Mass spectrometry data were integrated for 10 min, the corresponding lower limit of detection (LOD) based on three standard deviations of the background noise was estimated to be lower than 5 × 10 3 molecules cm −3 ; for the statistical analysis presented in Fig. 2 , values below the LOD were replaced by LOD/ \(\root {2} \of {2}\) [57] . For a detailed description of the instrument, see Jokinen et al. [12] , and for a detailed analysis of HIO 3 detection with a nitrate CIMS the reader is referred to Sipilä et al. [21] . The chemical composition of naturally charged negative ions was measured with an APi-TOF, this is the same mass spectrometer described before but without a chemical ionization unit. For a description of the instrument see Junninen et al. [11] . The absolute transmission of the APi-TOF was not characterized, therefore measurements are reported in counts per second (cps) and cannot be converted into atmospheric concentrations. The size distribution of ions and particles below 40 nm was measured with a NAIS [58] . The aerosol size distribution was measured with a scanning mobility particle sizer, range 18–660 nm, and with a differential mobility particle sizer (DMPS), range 10–959 nm, both instruments were custom made [59] , [60] . A TSI condensation particle counter (CPC) 3776 and a particle size magnifier (PSM) were used to measure the total particle concentration above 2.5 nm. The PSM was not able to measure particles below 2.5 nm because of issues with the saturator flow but overall it compared very well with the UCPC [61] . The UFP time series in Fig. 2b was obtained by combining measurements from both the CPC3776 and the PSM [62] . The particle size distribution shown in Fig. 4a was obtained combining measurements from the NAIS and the DMPS [63] . A comparison of the NAIS with the DMPS and the UCPC data is reported in Supplementary Note 1 and Supplementary Figs. 11 and 12 . Cloud residuals were sampled using a ground-based counterflow virtual impactor (CVI) inlet. The working principles of the CVI inlet are described in detail in Shingler et al. [64] . The ground-based version uses a wind tunnel to accelerate air onto the tip of the inlet, where the counterflow prevents non-activated aerosol (particles with low inertia) from entering the sample flow but allows cloud droplets and ice crystals pass through. The droplet/crystal cut size depends on the flow rates in the inlet, and was around 7.8 µm (aerodynamic diameter) with our set-up. The geometry of the CVI inlet and the difference between the wind tunnel airspeed and the sample flow rate result in the sample volume being enriched in cloud particles compared to the ambient air. Concentrations measured behind the CVI inlet therefore have to be divided by an enrichment factor, which can be calculated from the aforementioned parameters (see Shingler et al. [64] ). The enrichment factor was around 6.5 during the Arctic Ocean 2018 campaign. The cloud residual size distributions were not corrected for the droplet sampling efficiency of the CVI inlet, since the forward scattering spectrometer probe (FSSP) was not working for the event discussed in this paper. Cloud residual concentrations and number size distributions were measured with a TSI CPC3772 and a custom made DMPS in the size range 17–959 nm. CCN measurements were performed using a commercial DMT CCN counter scanning at five different SSs (0.1%, 0.2%, 0.3%, 0.5%, and 1.0%) [65] . All particle number measurements were corrected for diffusion and impaction losses using either the particle loss calculator [66] or user-made scripts based on the same equations. Ozone measurements were performed using a model 205 ozone monitor from 2BTechnologies [67] . The instrument was calibrated after the campaign and the data were corrected for a baseline drift based on zero measurements before and after the expedition. The overall accuracy of the instrument is estimated to be within 5% of the reading. All gas and aerosol measurements were cleaned from ship pollution using an algorithm based on the derivative of the ultrafine particle concentration, the PSD, CO 2 , black carbon measurements as well as wind direction [68] . The surface mixed layer height was estimated from the temperature profile measured from radiosondes which were launched every 6 h [69] . The surface inversion was calculated according to the algorithm from Tjernström and Graversen [70] . Data were linearly interpolated between each radiosonde. We adjusted the surface mixed layer height at noon on 17 September based on an inspection of the temperature profile that revealed a first inversion at 90 m. The algorithm did not identify this inversion because the temperature was not monotonically increasing. The dry deposition velocity can be calculated as the inverse of the sum of the aerodynamic, the quasi-laminar and the canopy resistance [71] . We assumed a neutral boundary layer to calculate the aerodynamic resistance and used the sulfuric acid diffusion coefficient to calculate the quasi-laminar resistance. The canopy resistance over snow surfaces is generally assumed to be equal to zero [71] ; hence, we did not consider it. Both the aerodynamic and the quasi-laminar resistance depends on the inverse of the friction velocity which can be calculated from wind speed [71] . Using the wind speed measurements from the ship, we have derived a dry deposition velocity time series whose median and IQR are 0.67 [0.39–0.96] cm s −1 . These values are comparable to the nitric acid dry deposition velocity measured in Svalbard [72] . The 10-day backward trajectories were calculated by Heini Wernli (ETH Zürich, Switzerland) using the Lagrangian analysis tool LAGRANTO and wind fields from 3-hourly operational ECMWF analyses, interpolated to a regular grid with 0.5° horizontal resolution on the 137 model levels [73] . The meteorological data were collected from a weather station installed on the 7th deck of the I/B Oden at ~25 m above sea level [74] . The majority of the data were processed using Python and in particular Scipy, Pandas, and Numpy libraries [75] , [76] , [77] , the raw mass spectrometer data were treated using Matlab and the TofTool library [11] . All the plots were produced using Matplotlib [78] . NPF events We identified 11 NPF events during our campaign, four of which were reported already in the main text (one event in Fig. 1a and three events in Fig. 3a ). The remaining events are shown in Supplementary Fig. 2 by means of the corresponding particle and negative-ion size distribution. When available the sulfuric and HIO 3 concentration is also reported. Different events are marked with a Roman numeral. We excluded from this list two events that were heavily influenced by pollution (on 12 and 26 August) and another event that occurred at the beginning of the campaign while we were still in the marginal ice zone. We used a different color map (i.e. magma instead of viridis) to highlight periods that were potentially influenced by the ship pollution for more than 10 min. Shorter pollution periods were not included because these are spikes associated with short events (e.g. a helicopter flight) that do not affect the overall aerosol population. Seasonal variation and background aerosol concentration We report seasonal variations of the three major acids, i.e. sulfuric acid, HIO 3 , and MSA, detected with the nitrate CIMS in Supplementary Fig. 3 . We used 27 August as the dividing date between summer and autumn based on the start of the freeze-up period as explained in the main text. All the three compounds show higher concentrations during autumn compared to summer, however, HIO 3 is characterized by the largest increase in both relative and absolute terms. The iodic acid median concentration is more than five times higher in autumn compared to summer, whereas sulfuric acid and MSA show less than a twofold increase. The same figure illustrates also the seasonal increase in the concentration of UFP particles, whose median concentration is 12 times higher in autumn compared to summer. Although the sulfuric acid concentration is much lower compared to HIO 3 these two species are correlated on the short-term scale (see for example, Fig. 3b ). This correlation is explained by the very short lifetime of these two acids whose concentration is largely controlled by changes in the sinks (i.e. fog or particle condensation as explained in the Iodic acid sources, sinks and variability section). We have analyzed back-trajectories to investigate whether the seasonal change could be related to a different air mass source regions. However, there is no evidence for a systematic shift in the air mass origin as shown in Supplementary Fig. 4 . We considered only trajectories in the boundary layer for 5 days before arriving at the ship position. The extremely low aerosol background concentration is shown in Supplementary Fig. 5 as a box and whiskers plot for concentrations of particles with a diameter larger than 30 nm, CCN concentrations at 0.3% SS and the sulfuric acid CS [79] . Iodic acid model We assume that HIO 3 is entirely produced by iodine that is emitted as I 2 to the atmosphere at a rate E* [molecules cm −2 s −1 ] and photolysed at a rate J [s −1 ]: 
    [ dI_2/dt = E^ ∗/h - J[ I_2] = 0, ]
 (2) 
    [ [ I_2] = E^ ∗ /h/J, ]
 (3) with h being the height of the surface mixed layer. The HIO 3 concentration can be described by 
    [ d[ HIO_3]/dt = 2J[ I_2] - v_d/h[ HIO_3] - CS[ HIO_3] = E/h - ( v_d/h - CS)[ HIO_3], ]
 (4) with E = 2 E * being the emission rate in terms of iodine atoms cm −2 s −1 . In a steady state, this equation reduces to 
    [ [ HIO_3] = E/v_d + h ·CS→log _10( [ HIO_3]) = log _10E - log _10( v_d + h ·CS). ] (5) From Eq. ( 5 ) it follows that, for a given emission factor E , the logarithm of the HIO 3 concentration should vary linearly with the logarithm of \(- (v_{\rm{{d}}} + h \cdot {\rm{{CS}}})\) with a unity slope. Equation ( 5 ) can be used to infer the emission factor E for periods of data where the steady-state assumption holds. We identified periods of steady state by looking at the derivatives of both the HIO 3 and the \((v_{\rm{{d}}} + h \cdot {\rm{{CS}}})\) signals over their respective time series and considered only those periods where the derivative to signal ratio was below 5% for both. An exception was made when only one or two data points were exceeding the 5% threshold. We only considered periods longer than 90 min in order to obtain enough data. Before calculating the derivative we smoothed the data with a one-hour running average and a hamming type window to reduce instrumental noise that would be amplified by the derivative calculation. With this approach, we identified 11 steady-state periods as shown in Fig. 2e . We estimated the emission factor of each individual data point [80] of these periods following Eq. ( 5 ) and show the distribution of these values in Supplementary Fig. 6 . Another way to investigate the applicability of this model to our dataset is to integrate numerically Eq. ( 4 ) and simulate the evolution of HIO 3 . The model does not include losses of HIO 3 to cloud droplets and so HIO 3 could be simulated only for periods without fog. In Supplementary Fig. 7 we report the simulation results for two periods corresponding to two different emission rate scenarios. We have used a simple Euler integration method to simulate the HIO 3 evolution and initialized it with the mean HIO 3 concentration in the first hour. The simulation was run with three different emission factors to highlight the sensitivity of the result on the emission. In the first simulation, the model is able to reproduce the measurements fairly well and starts deviating from its initialization only after about 14 h (around 12:00). As expected, it does not reproduce the rapid decrease of HIO 3 due to scavenging in fog after 13:00. In the second simulation, the model captures the overall trend but the discrepancy with the measurements is higher. There is, for example, a rapid change in the HIO 3 concentration after 06:00 which is not captured by the model. This is probably due to a sudden change in the air mass (see also the PSD of event V in Supplementary Fig. 2 ). The model incorporates the iodine emission and its conversion into HIO 3 into this E factor. Because the HIO 3 production pathways is still not fully understood [43] , it is not possible to estimate a real iodine flux based on our measurements. Moreover, E represents a lower limit estimate of the real iodine flux given that only a fraction of the emitted iodine atoms would be converted to HIO 3 . However, the E factor range (Supplementary Fig. 6 ) provided in this study could be directly used by atmospheric models to simulate the HIO 3 concentration over the pack ice and estimate its role in terms of NPF. Fog scavenging Given the extremely low aerosol background the main sink for UFP over the central Arctic Ocean is scavenging by coagulation in fog and cloud droplets. In a mid-latitude non-precipitating cloud the lifetime of a 10-nm particle would be about 11 min [71] . However, Arctic clouds are typically characterized by a lower droplet number because of the CCN limitation and this has an effect on the UFP lifetime. Hence, we have calculated the aerosol lifetime starting from the average droplet size distribution measured using an FSSP during MOCCHA [81] . We included all data until 5 September as the instrument broke down afterwards. In Supplementary Fig. 8b we show the corresponding median and IQR droplet number size distribution. In Supplementary Fig. 8a we report the estimated lifetime of an interstitial aerosol particle as a function of its size (only losses due to coagulation into fog droplets are included). In this case the lifetime of a 10-nm particle would be about 10 h. The difference in lifetime for a representative Arctic and mid-latitude cloud is striking but consistent with the large difference in droplet number concentration (generally <30 cm −3 in the central Arctic Ocean and about 1000 cm −3 in a mid-latitude cloud [71] ). In the same figure, we highlight the lifetime of HIO 3 , considered as a 0.5-nm particle, which is around 2 min. The diameter is calculated using HIO 3 bulk properties, i.e. density and mass. This value is consistent with the HIO 3 decay time in fog and is much lower compared to a situation where the lifetime was controlled by condensation on pre-existing aerosol only (Supplementary Fig. 5 ). Spatial extent of NPF events A simple estimate for the spatial extent of an NPF event can be calculated assuming a homogeneous air mass over the entire event duration: 
    L = W_sΔt,
 (6) with ∆ t being the duration of the event, W s the mean wind speed during the event, and L the air mass diameter. This is a lower limit estimate because it is based on the assumption that the measurement location was sitting at the edge of the air mass at the beginning of the event. Applying such a calculation to the NPF event of 5 September leads to an areal diameter of about 160 km. Growth rate calculation and modeling We calculated the growth rate using the mode diameter fitting procedure. The data obtained from the NAIS were averaged to 10 min and the PSD was fitted with a multi-modal lognormal distribution. Other methods such as the appearance time-based calculation did not work reliably due to air mass inhomogeneity which produced fluctuations in the particle number concentration [82] . The growth rate was calculated only for those periods showing a continuous growth for at least 2 h excluding periods influenced by fog, clear air mass changes or the ship exhaust. For example we did not calculate a growth rate for the 6 September event (Fig. 3a ) because a mix of pollution, fog, and air mass inhomogeneity impeded the identification of a clearly growing mode. We used a hard-sphere model based on kinetic condensation to estimate the contributions by sulfuric and HIO 3 to the growth [44] . This model requires knowledge of the condensing vapor volumes which can be inferred from their bulk-phase densities. However, the molecular volume depends on the degree of hydration, which in principle is not known because it is not measured directly by the mass spectrometer. Considering that the median and [IQR] of the relative humidity during MOCCHA were 95.7% and [90.8−98.4]%, the degree of hydration is expected to be high and should not be neglected. Quantum chemical calculations for sulfuric acid predict each molecule to be prevalently bound to three water molecules at 80% RH, therefore we took this value as a lower limit estimate and calculated the sulfuric acid–water solution density accordingly [83] , [84] . Concerning HIO 3 , there are no studies reporting the hydrate distribution at ambient relevant RH. Khanniche et al. [85] showed that HIO 3 forms stable hydrates with up to two water molecules but did not investigate larger hydrates. It has also been suggested that the iodate dimer (HIO 3 IO 3 − ) is hydrated with up to 5 water molecules at 65% RH [86] . Therefore, we assumed the HIO 3 monomer to be prevalently bound to three water molecules and estimated its volume based on bulk-phase density measurements [87] . This is in analogy with the sulfuric acid case and reasonable given the high RH values experienced during MOCCHA. Finally, the mass diameter was converted into a mobility diameter adding 0.3 nm as suggested by Larriba et al. [88] The sulfuric acid growth rate EF was derived from Stolzenburg et al. [45] and applied also to the HIO 3 growth. This EF is based on a mechanism driven by van-der-Waals forces between UFP and neutral molecules and depends on the condensing species. HIO 3 will certainly have a different EF compared to sulfuric acid, however this value is not known and the two molecules share similar properties (e.g. dipole moment), therefore, we expect the final EF to be similar. Critical diameter calculations In Supplementary Fig. 9 we report critical diameter calculations at three different SSs (0.2%, 0.3%, and 1.0%) based on CCN measurements. The critical diameter is calculated assuming an internally mixed aerosol population and integrating the particle number concentration downward from the largest diameter of the aerosol number size distribution [48] . It is important to note the period from 09:00 until 12:00 which is characterized by fog without accumulation mode particles (see Fig. 4 in main text). The comparison between the cloud residual number concentration and the dry aerosol distribution suggests that particles with a diameter as small as 37 nm were activating. This value is consistent with the critical diameter at 1% SS. Comparison with aerosol iodine concentration at Alert An increase in the concentration of iodine in autumn based on aerosol measurements was shown for the first time by Sirois and Barrie [52] more than 20 years ago. More recently, Sharma et al. [38] extended the analysis up to 2006 confirming the existence of an iodine autumn peak. Their data are based on instrumental neutron activation analysis (INAA) of aerosol filters collected at Alert, Canada (82.5°N 62.3°W) by the Canadian Aerosol Baseline Measurement (CABM) Network, Climate Research Division, Environment and Climate Change Canada from 1981 until 2006. In Supplementary Fig. 10 we compare weekly mean HIO 3 absolute concentrations in the gas phase from our measurements and iodine in the aerosol phase from Sharma et al. [38] The agreement between these two datasets is remarkable considering that they are from two locations about 900 km apart, from different decades and obtained with different measurement techniques. Besides the similar time trends only a few hours of condensation of the available HIO 3 on pre-existing particles is required to reach the observed concentrations of iodine in the aerosol at Alert. The key message is that our observations are not limited to a single year and specific location in the Arctic but have likely been observed over multiple decades and are representative for the high Arctic. Sharma et al. [38] also showed that the aerosol iodine autumn concentration did not vary significantly from 1981 to 2006, indicating that the iodine emission rate has been relatively stable for the last few decades. This observation is different from recent results that reported almost a doubling of the atmospheric iodine concentration from 1980 to 2010 in the North Atlantic [89] . It is not the scope of this work to investigate the differences between these two previous studies, however, considering the similarities of our results with those reported in Sharma et al. [38] it seems likely that the autumn iodine emissions in the central Arctic Ocean did not change significantly during the past few decades.